Heteroepitaxial vertical perovskite hot-electron transistors down to the monolayer limit 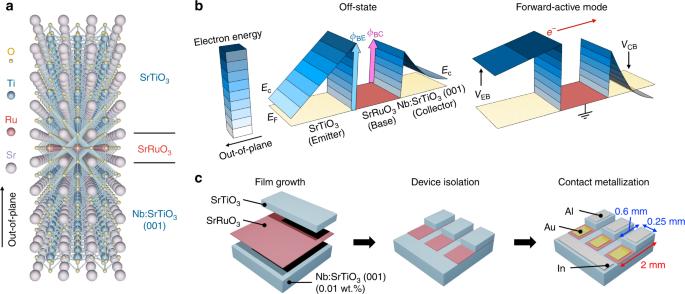Fig. 1 Schematics and working principle of the perovskite hot-electron transistor (HET).aThe crystal structure of the atomically thin HET with a SrTiO3emitter/SrRuO3base/Nb:SrTiO3(001) collector trilayer.bSchematic illustration of the HET energy band diagram in the off-state (left) and in the common-base forward-active mode (right). In device operation, hot electrons are injected across the forward-biased base–emitter (BE) junction, traverse across the grounded base, and are collected across the reverse-biased base–collector (BC) junction.cDevice process flow of the HET with laterally staggered electrical contacts. Two-dimensional heterostructures combined with vertical geometries are candidates to probe and utilize the physical properties of atomically-thin materials. The vertical configuration enables a unique form of hot-carrier spectroscopy as well as atomic-scale devices. Here, we present the room-temperature evolution of heteroepitaxial perovskite hot-electron transistors using a SrRuO 3 base down to the monolayer limit ( ∼ 4 Å). As a fundamental electronic probe, we observe an abrupt transition in the hot-electron mean free path as a function of base thickness, coinciding with the thickness-dependent resistive transition. As a path towards devices, we demonstrate the integrated synthesis of perovskite one-dimensional electrical edge contacts using water-soluble and growth-compatible Sr 3 Al 2 O 6 hard masks. 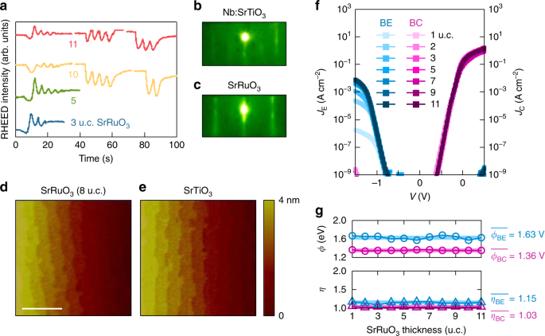Fig. 2 Heterostructure fabrication and room-temperature junction characteristics.aRHEED intensity oscillations for the growth of SrRuO3base. In situ RHEED patterns ofbNb:SrTiO3(001) andcSrRuO3. AFM topographies ofd8 unit cell (u.c.) SrRuO3, andeSrTiO3thin films, showing a clear perovskite step-and-terrace surface structure. The scale bar is 1 μm.fCurrent-voltage characteristics of the BC and BE Schottky junctions, for various SrRuO3thicknesses down to the monolayer limit.gExtracted BC and BE junction Schottky barrier heightϕ(top) and ideality factorη(bottom). The solid lines are the mean values. 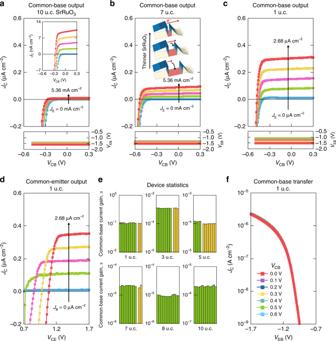Fig. 3 Room-temperature electrical characterization of variable thickness SrRuO3HETs. Common-base output characteristics (top) and voltage feedback (bottom) for SrRuO3thicknesses ofa10 u.c. andb7 u.c., asJEis increased from 0 to 5.36 mA cm−2, in 1.34 mA cm−2steps; andc1 u.c., asJEis increased from 0 to 2.68 μA cm−2, in 0.67 μA cm−2steps. The inset toashows the region where clear transconductance can be seen for 10 u.c. SrRuO3thickness. The inset tobshows a schematic illustration of the increase of hot-electron transfer as the base becomes thinner. The constant voltage feedback curves in the common-base output characteristics demonstrate the complete electrostatic screening by the base metal.dCommon-emitter output characteristics for 1 u.c. SrRuO3thickness, asJBis increased from 0 to 2.68 μA cm−2, in 0.67 μA cm−2steps.eDevice statistics on common-base current gainα. For a specified SrRuO3thickness, each bar represents a single device and each color represents a distinct sample from a different fabrication run.fCommon-base transfer characteristics for 1 u.c. SrRuO3thickness withVCBranging from 0.0 to 0.6 V, in 0.1 V steps.VEBrequired for the onset ofJCis independent ofVCB, indicating pure HET operation. Edge-contacted monolayer-base transistors exhibit on/off ratios reaching ∼ 10 8 , complete electrostatic screening by the base manifesting pure hot-electron injection, and excellent scaling of the output current density with device dimensions. These results open new avenues for incorporating emergent phenomena at oxide interfaces and in heterostructures. Along with exfoliated two-dimensional (2D) materials [1] , [2] , [3] , [4] , [5] , atomic-scale artificial perovskite oxide heterostructures offer exciting opportunities [6] , [7] for new devices and experimental probes of quantum materials. Specifically, designing vertical architectures incorporating these materials has unique advantages. It effectively utilizes their atomically thin nature by actively setting the channel length to an atomic scale, which would be an enabling pathway for fast electronics [8] , which is technically challenging in planar devices. More importantly, the perpendicular geometry can diversify functionalities in fundamental studies and applications by integrating layers with a wide range of physical properties in an interface-specific manner. For example, hot-electron transport across interfaces can be used to surpass fundamental thresholds [9] , [10] , such as the thermodynamic Shockley–Queisser limit in solar cells. In oxide heterostructures, hot-electron spectroscopy [11] would be an invaluable tool to investigate the nanometer scale electronic reconstructions that are often observed at interfaces and in confined geometries [7] . In pursuit of this approach, we demonstrate the evolution of a highly robust vertical hot-electron transistor (HET) [12] based on perovskite oxide heterostructures down to the monolayer-base limit, consisting of a SrTiO 3 emitter (both Nb-doped and undoped), atomically thin SrRuO 3 base, and Nb:SrTiO 3 (001) collector (Fig. 1 ; see the Methods section). Fig. 1 Schematics and working principle of the perovskite hot-electron transistor (HET). a The crystal structure of the atomically thin HET with a SrTiO 3 emitter/SrRuO 3 base/Nb:SrTiO 3 (001) collector trilayer. b Schematic illustration of the HET energy band diagram in the off-state (left) and in the common-base forward-active mode (right). In device operation, hot electrons are injected across the forward-biased base–emitter (BE) junction, traverse across the grounded base, and are collected across the reverse-biased base–collector (BC) junction. c Device process flow of the HET with laterally staggered electrical contacts. Full size image Heterostructure fabrication and junction characteristics In device operation, hot electrons are injected out-of-plane across the forward-biased base–emitter (BE) junction, traverse the grounded base, and are collected across the reverse-biased base–collector (BC) junction. We first focus on devices with conventional laterally staggered surface contacts. The heteroepitaxial trilayer shows epitaxial and atomically flat surface topographies with the perovskite step-and-terrace structure of the underlying substrate, as seen by atomic force microscopy (AFM) and reflection high-energy electron diffraction (RHEED) patterns (Fig. 2a–e ). Accordingly, both interfaces form Schottky junctions following the thermionic emission model, evident from the rectifying current-voltage characteristics with constant Schottky barrier height ϕ and ideality factor η near unity down to the monolayer limit (Fig. 2f, g ). This is remarkable considering that only a single unit cell (u.c.) of SrRuO 3 ( ∼ 4 Å) is responsible for the Schottky junction formation at both interfaces. Fig. 2 Heterostructure fabrication and room-temperature junction characteristics. a RHEED intensity oscillations for the growth of SrRuO 3 base. In situ RHEED patterns of b Nb:SrTiO 3 (001) and c SrRuO 3 . AFM topographies of d 8 unit cell (u.c.) SrRuO 3 , and e SrTiO 3 thin films, showing a clear perovskite step-and-terrace surface structure. The scale bar is 1 μm. f Current-voltage characteristics of the BC and BE Schottky junctions, for various SrRuO 3 thicknesses down to the monolayer limit. g Extracted BC and BE junction Schottky barrier height ϕ (top) and ideality factor η (bottom). The solid lines are the mean values. Full size image Electrical characteristics of variable thickness SrRuO 3 HETs The common-base and common-emitter output characteristics of these devices show clear transconductance down to the monolayer limit (Fig. 3a–d ). As the base becomes thinner, more hot electrons overcome ϕ BC due to less scattering in the base; accordingly, the collector current density J C increases exponentially (Fig. 3b , inset). In general, an atomically thin base could be prone to the formation of pinhole and edge defects which electrostatically couple the emitter and the collector via a semiconducting channel, inducing permeable-base transistor operation [13] , [14] governed by the drift-diffusive transport of Fermi-level electrons, as opposed to hot-electron transport. To rule out this possibility, we demonstrate that the metal base in our HETs completely screens the electric field and electrically isolates the emitter and the collector, by the measurement of constant voltage feedback curves (Fig. 3a–c ). Fig. 3 Room-temperature electrical characterization of variable thickness SrRuO 3 HETs. Common-base output characteristics (top) and voltage feedback (bottom) for SrRuO 3 thicknesses of a 10 u.c. and b 7 u.c., as J E is increased from 0 to 5.36 mA cm −2 , in 1.34 mA cm −2 steps; and c 1 u.c., as J E is increased from 0 to 2.68 μA cm −2 , in 0.67 μA cm −2 steps. The inset to a shows the region where clear transconductance can be seen for 10 u.c. SrRuO 3 thickness. The inset to b shows a schematic illustration of the increase of hot-electron transfer as the base becomes thinner. The constant voltage feedback curves in the common-base output characteristics demonstrate the complete electrostatic screening by the base metal. d Common-emitter output characteristics for 1 u.c. SrRuO 3 thickness, as J B is increased from 0 to 2.68 μA cm −2 , in 0.67 μA cm −2 steps. e Device statistics on common-base current gain α . For a specified SrRuO 3 thickness, each bar represents a single device and each color represents a distinct sample from a different fabrication run. f Common-base transfer characteristics for 1 u.c. SrRuO 3 thickness with V CB ranging from 0.0 to 0.6 V, in 0.1 V steps. V EB required for the onset of J C is independent of V CB , indicating pure HET operation. Full size image The common-base transfer characteristics further corroborate this complete screening in the base by showing that the V EB required for the onset of J C is independent of V CB (Fig. 3f ). Considering the Thomas–Fermi screening length L TF of ∼ 2 Å in SrRuO 3 at both interfaces, it is significant that the transistor still operates as a pure HET with only a single u.c. of SrRuO 3 . The monolayer common-base current gain α ∼ 0.12 and common-emitter current gain β ∼ 0.14 follow the expected relation β = α /(1– α ). After optimizing the processing conditions, our devices show 100% HET yield with exceptionally high stability and reproducibility for >100 devices examined (Fig. 3e ). This is in contrast to prior work using a manganite base with low HET yield and dominantly permeable-base devices [14] . We attribute this important difference to the perfect registry of SrRuO 3 with the underlying substrate; namely, the common Sr cation throughout the trilayer, with interfaces free of polar electrostatic boundary conditions [15] , [16] . Probing the fundamental characteristics of hot electrons The extremely high reliability of these HETs allows the experimental determination of hot-electron parameters, which were not previously accessible due to low yield and device-to-device fluctuations [14] . As shown in Fig. 4a–c , we observe the systematic thickness-dependent evolution of α over a wide range of ∼ 7 orders of magnitude. Note that these devices were optimized for stability, not output current density, by incorporating a thick undoped SrTiO 3 emitter (Fig. 1 ). This avoided the growth-to-growth carrier density fluctuations of doped SrTiO 3 , which would obscure the intrinsic response for thicker SrRuO 3 . The exponential trend of α can be parametrized by the hot-electron mean free path λ H as [12] 
    α = {[                                α _0 ×exp(-t/λ _H,I),                                           t ≤ 3 u.c. ; α _0 ×exp(-3  u.c./λ _H,I) ×exp[-(t-3 u.c. )/λ _H,B],                                    t    >    3  u.c. ].,
 (1) where t is the SrRuO 3 thickness, α 0 is α extrapolated to t = 0 u.c., and λ H,B ( λ H,I ) is the bulk (interfacial) hot-electron mean free path. The fact that α fits very well the exponential form self-consistently confirms HET operation, and highlights the ability to control SrRuO 3 thickness on the atomic level. These results indicate that SrRuO 3 is homogeneous with λ H,I ∼ 0.3 ± 0.01 u.c. up to 3 u.c. However, two distinct regions exist for thicker SrRuO 3 : the interfacial region with λ H,I , and the ‘bulk’ region away from the interface with λ H,B ∼ 1.4 ± 0.03 u.c., in good correspondence to recent studies using ballistic electron emission microscopy across the vacuum/SrRuO 3 interface [17] . Fig. 4 Probing the fundamental characteristics of hot electrons down to the monolayer limit of the HET at room temperature. Common-base transfer characteristics for different SrRuO 3 thicknesses at V CB = 0 V, plotted as a V EB versus J C , and b J E versus J C . c Common-base current gain α (red open circles) at V CB = 0 V and in-plane conductivity σ of the SrRuO 3 /SrTiO 3 (001) heterostructures (blue open circles) as a function of SrRuO 3 thickness at room temperature. α spans a wide range of ~7 orders of magnitude and self-consistently follows an exponential trend, illustrating the HET operation of the devices. Two distinct exponential regimes exist as a function of SrRuO 3 thickness, where the deduced hot-electron mean free path λ H is ~0.3 ± 0.01 u.c. from the data up to 3 u.c., and ~1.4 ± 0.03 u.c. from the data for thicker base. Below 3 u.c., fractional coverage devices smoothly interpolate. The red solid lines are best linear fits to the two regimes. d λ H near the center of the SrRuO 3 base layer (red solid line) and Fermi-electron mean free path λ F (blue open circles) as a function of SrRuO 3 thickness. The quasi-universal thickness-dependent metal–insulator transition is evident both from λ H and λ F across the same critical thickness. The blue solid line is a fit assuming a dominant surface/interface scattering (see text). The inset shows the thickness-dependent in-plane resistivity ρ as a function of temperature T for SrRuO 3 /SrTiO 3 (001) heterostructures. Full size image The abrupt transition in λ H at 3 u.c. is quite reminiscent of the commonly observed resistivity transition for ultrathin SrRuO 3 [18] , [19] , [20] , [21] . While there are some variations in the observed critical thickness, and debate on its origin, we see the same transition in our films. 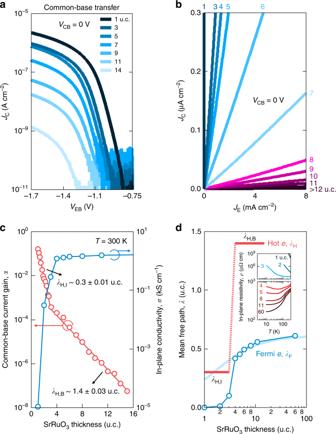Fig. 4 Probing the fundamental characteristics of hot electrons down to the monolayer limit of the HET at room temperature. Common-base transfer characteristics for different SrRuO3thicknesses atVCB= 0 V, plotted asaVEBversusJC, andbJEversusJC.cCommon-base current gainα(red open circles) atVCB= 0 V and in-plane conductivityσof the SrRuO3/SrTiO3(001) heterostructures (blue open circles) as a function of SrRuO3thickness at room temperature.αspans a wide range of ~7 orders of magnitude and self-consistently follows an exponential trend, illustrating the HET operation of the devices. Two distinct exponential regimes exist as a function of SrRuO3thickness, where the deduced hot-electron mean free pathλHis ~0.3 ± 0.01 u.c. from the data up to 3 u.c., and ~1.4 ± 0.03 u.c. from the data for thicker base. Below 3 u.c., fractional coverage devices smoothly interpolate. The red solid lines are best linear fits to the two regimes.dλHnear the center of the SrRuO3base layer (red solid line) and Fermi-electron mean free pathλF(blue open circles) as a function of SrRuO3thickness. The quasi-universal thickness-dependent metal–insulator transition is evident both fromλHandλFacross the same critical thickness. The blue solid line is a fit assuming a dominant surface/interface scattering (see text). The inset shows the thickness-dependent in-plane resistivityρas a function of temperatureTfor SrRuO3/SrTiO3(001) heterostructures. 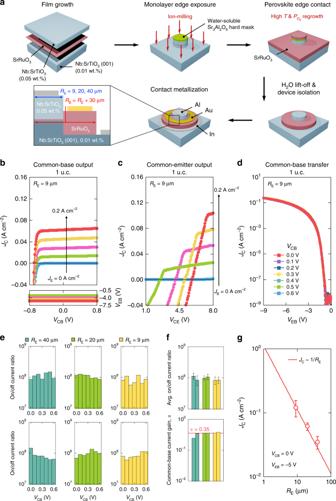Fig. 5 Room-temperature electrical characterization of monolayer-base HETs with a perovskite one-dimensional electrical edge contact.aSchematic of the perovskite edge contact fabrication process using a water-soluble and growth-compatible Sr3Al2O6hard mask layer30.RE(RB) is the emitter (base) radius.bCommon-base output characteristics (top) and voltage feedback (bottom), asJEis increased from 0 to 0.2 A cm−2, in 0.05 A cm−2steps.cCommon-emitter output characteristics, asJBis increased from 0 to 0.2 A cm−2, in 0.05 A cm−2steps.dCommon-base transfer characteristics withVCBranging from 0.0 to 0.6 V, in 0.1 V steps.REis 9 μm for the devices shown inbthroughd.eOn/off current ratio as a function ofVCBranging from 0.0 to 0.6 V, in 0.1 V steps. Each panel represents a different device.fOn/off current ratio averaged overVCBranging from 0.0 to 0.6 V (top) and common-base current gainα(bottom) for devices shown ine. The red solid line representsα= 0.35, each bar represents a different device, and the error bars represent the standard deviations. The blue, green, and yellow solid bars ineandfrepresent devices withRE= 40, 20, and 9 μm, respectively.gJCas a function ofREatVCB= 0 V andVEB= −5 V. The error bars represent the standard deviations. The data (red open circles) self-consistently scale with the residual base resistance underneath the emitter asJC~ 1/RE(red solid line)31. Figure 4c shows the thickness-dependent evolution of the room-temperature in-plane conductivity for identically grown samples on an undoped substrate. Notably, for 3 u.c. and below, the temperature dependence is insulating, while for 4 u.c. and above, increasingly bulk-like metallic temperature dependence is observed (Fig. 4d , inset). From a fundamental perspective, λ H has a rather interesting comparison to that for conventional transport, λ F , the Fermi-electron mean free path. λ F can be estimated from the resistivity ρ , which can be expressed via Boltzmann transport as \(\rho = 3{\uppi}^2\hbar /q^2k_{\mathrm{F}}^2\lambda _{\mathrm{F}}\) , where ħ is the reduced Planck’s constant, q is the elementary charge, and k F is the Fermi wave vector [22] . Figure 4d shows the deduced thickness-dependent λ F at room temperature. As previously noted, the smooth decrease of λ F down to 4 u.c. arises from enhanced surface/interface scattering [20] . Even in the atomistically clean limit, surface/interface scattering impacts the in-plane transport of ultrathin films [23] , including diffuse scattering at step edges, whereby λ F can be expressed in terms of t using Matthiessen’s rule as \({\mathrm{1}}/\lambda _{\mathrm{F}} = 1/\lambda _{{\mathrm{F,B}}} + 1/t_0t\) , where λ F,B is the bulk Fermi-electron mean free path, and t 0 is the surface/interface scattering constant. Estimating λ F,B as λ F for t = 60 u.c., λ F fits well this functional form down to 4 u.c. but then drastically decreases in the thinner films with insulating temperature dependence. As has been previously emphasized, the extremely short λ F,B (300 K) ∼ 0.6 u.c. in SrRuO 3 is highly inconsistent with coherent transport in conventional metals [22] , [24] , and this ‘badly metallic’ behavior is a characteristic feature of strongly correlated metals under much current investigation [25] . Here we find that λ H,B exceeds our estimate for λ F,B by a factor of ∼ 2.3 (Fig. 4d ). This enhancement could originate from Ru 4 d electrons effectively screening the inelastic electron–electron scattering of hot electrons [26] . Note that λ H,B can be isolated from surface/interface scattering, as indicated by its constant thickness dependence above the sharp transition between 3 u.c. and 4 u.c.—this is a unique advantage of these thickness-dependent hot-electron experiments, enabling a direct measure of fundamental scattering mechanisms without surface/interface contributions. The surprising enhancement of λ H,B with respect to λ F,B suggests that further hot-electron spectroscopic studies of strongly correlated metals would provide valuable insights in this relatively unexplored regime. Perovskite one-dimensional electrical edge contacts We turn now to considerations relevant for the potential development of monolayer heterostructures for practical devices. While there are several important issues that need to be addressed, a central obstacle is the low output current density in the HETs presented thus far ( J C ∼ μA cm −2 ). Two significant contributions are the high emitter resistance introduced via thick undoped SrTiO 3 (needed for device stability investigating the thick-base regime, but which limits hot-electron injection), and the in-plane base series resistance arising from the laterally staggered contact geometry, which becomes increasingly dominant in the monolayer limit. In order to address these issues, we can thin down and dope the emitter, which readily improves the emitter resistance by orders of magnitude [15] , [27] , [28] . Furthermore, we demonstrate here the synthesis of a perovskite one-dimensional electrical edge contact, in analogy to that recently developed for 2D materials [29] , using a water-soluble and growth-compatible Sr 3 Al 2 O 6 hard mask layer [30] (Fig. 5a ; see the Methods section). The Sr 3 Al 2 O 6 layer not only bypasses aggressive lift-off processes, but also is stable at high growth temperatures and oxidizing conditions, allowing for the corresponding growth of the perovskite edge contact. Fig. 5 Room-temperature electrical characterization of monolayer-base HETs with a perovskite one-dimensional electrical edge contact. a Schematic of the perovskite edge contact fabrication process using a water-soluble and growth-compatible Sr 3 Al 2 O 6 hard mask layer [30] . R E ( R B ) is the emitter (base) radius. b Common-base output characteristics (top) and voltage feedback (bottom), as J E is increased from 0 to 0.2 A cm −2 , in 0.05 A cm −2 steps. c Common-emitter output characteristics, as J B is increased from 0 to 0.2 A cm −2 , in 0.05 A cm −2 steps. d Common-base transfer characteristics with V CB ranging from 0.0 to 0.6 V, in 0.1 V steps. R E is 9 μm for the devices shown in b through d . e On/off current ratio as a function of V CB ranging from 0.0 to 0.6 V, in 0.1 V steps. Each panel represents a different device. f On/off current ratio averaged over V CB ranging from 0.0 to 0.6 V (top) and common-base current gain α (bottom) for devices shown in e . The red solid line represents α = 0.35, each bar represents a different device, and the error bars represent the standard deviations. The blue, green, and yellow solid bars in e and f represent devices with R E = 40, 20, and 9 μm, respectively. g J C as a function of R E at V CB = 0 V and V EB = −5 V. The error bars represent the standard deviations. The data (red open circles) self-consistently scale with the residual base resistance underneath the emitter as J C ~ 1/ R E (red solid line) [31] . Full size image As a result, the monolayer-base devices improved significantly: J C increased by ∼ 5 orders of magnitude; on/off current ratios reached ∼ 100,000,000; and α increased threefold to ∼ 0.35, with a corresponding enhancement of β to ∼ 0.54 (Fig. 5 ). Pure HET operation is evident from the voltage feedback curves and the transfer characteristics as discussed previously (Fig. 5b, d ). Most importantly, we find that J C self-consistently scales with the residual base resistance underneath the emitter as 1/ R E ( R E is the emitter radius) [31] , which is very favorable to device downscaling (Fig. 5g ). This confirms that the perovskite edge contact effectively minimizes the base series resistance by placing the contact at the edge of the monolayer base/emitter interface, and should enable high current density in sub-micron devices. Furthermore, the edge contact method developed here should be broadly useful for a wide range of oxide heterostructure devices. Heterostructure fabrication and device processing The heteroepitaxial trilayer was fabricated using pulsed laser deposition with a 248 nm KrF excimer laser using TiO 2 -terminated Nb:SrTiO 3 (001) substrates (0.01 wt% Nb dopant concentration). SrRuO 3 base (1 u.c. to 15 u.c.) was grown in 100 mTorr O 2 . The base thickness was controlled on the atomic scale by monitoring the in situ RHEED oscillations, where one oscillation corresponds to a single u.c. Coherent RHEED oscillations throughout the growth indicate high quality layer-by-layer growth of the SrRuO 3 . In particular, the growth of SrRuO 3 is interrupted every 4 u.c. for thicker films so that the adatoms on the surface can sufficiently rearrange, and preserve the step-and-terrace structure of the underlying substrate, as indicated by the RHEED intensity recovery right after the interruption (Fig. 2a ). This preservation of the step-and-terrace structure is especially critical for SrRuO 3 , because it has been otherwise reported to adversely affect the transport properties [20] . A ∼ 60 nm-thick SrTiO 3 emitter was consecutively grown through a rectangular template mask in 1 mTorr O 2 . The substrate temperature was 700 °C during the entire growth. The SrRuO 3 /SrTiO 3 (001) heterostructure was fabricated under the same growth conditions. The SrTiO 3 /SrRuO 3 /Nb:SrTiO 3 (001) trilayer was then Ar-ion etched into rectangular shapes, and annealed in 760 Torr O 2 at 350 °C for 6 h to fill oxygen vacancies generated by Ar-ion etching. Rectangular Au and Al electrodes were deposited using e-beam evaporation on the base and emitter, respectively. Indium was ultrasonically soldered onto the collector. These electrodes form Ohmic contacts to each layer. Perovskite one-dimensional electrical edge contact ∼ 30 nm-thick Nb:SrTiO 3 (0.05 wt% Nb dopant concentration)/monolayer SrRuO 3 /Nb:SrTiO 3 (001) heteroepitaxial trilayer was grown using the same substrates and growth conditions as noted above (the emitter was grown without the use of a template mask). The key step is the growth of a water-soluble and growth-compatible Sr 3 Al 2 O 6 hard mask layer on the trilayer. The Sr 3 Al 2 O 6 hard mask layer bypasses aggressive lift-off processes and also serves as a mask during Ar-ion etching and perovskite edge contact regrowth processes involving high growth temperatures and oxidizing conditions. A ∼ 180 nm-thick Sr 3 Al 2 O 6 hard mask layer [30] was grown in lithographically patterned circular shapes in 5 × 10 −6 Torr O 2 at room temperature, and capped with a ∼ 60 nm-thick SrTiO 3 grown in 1 mTorr O 2 at room temperature to enhance its stability in the air. The trilayer covered with the Sr 3 Al 2 O 6 hard mask layer in circular shapes was Ar-ion etched to expose the edge of the monolayer base and annealed in 760 Torr O 2 at 350 °C for 6 h. A ∼ 30 nm-thick SrRuO 3 edge contact was consecutively grown in 100 mTorr O 2 at 700 °C. The entire structure was then immersed into room-temperature filtered de-ionized water to dissolve the Sr 3 Al 2 O 6 hard mask layer. For device isolation, the trilayer was Ar-ion etched into larger circular shapes and annealed in 760 Torr O 2 at 350 °C for 6 h. Electrodes were deposited on each layer as noted above. Characterization AFM images were acquired in tapping mode. All electrical measurements of the device were performed using a semiconductor parameter analyzer in DC mode at room temperature in ambient conditions. The in-plane transport measurements were conducted in a four-point geometry with Au contacts for SrRuO 3 films.